Crystallographic and spectroscopic characterization and reactivities of a mononuclear non-haem iron(III)-superoxo complex Mononuclear non-haem iron(III)-superoxo species (Fe III -O 2 −· ) have been implicated as key intermediates in the catalytic cycles of dioxygen activation by non-haem iron enzymes. Although non-haem iron(III)-superoxo species have been trapped and characterized spectroscopically in enzymatic and biomimetic reactions, no structural information has yet been obtained. Here we report the isolation, spectroscopic characterization and crystal structure of a mononuclear side-on ( η 2 ) iron(III)-superoxo complex with a tetraamido macrocyclic ligand. The non-haem iron(III)-superoxo species undergoes both electrophilic and nucleophilic oxidation reactions, as well as O 2 -transfer between metal complexes. In the O 2 -transfer reaction, the iron(III)-superoxo complex transfers the bound O 2 unit to a manganese(III) analogue, resulting in the formation of a manganese(IV)-peroxo complex, which is characterized structurally and spectroscopically as a mononuclear side-on ( η 2 ) manganese(IV)-peroxo complex. The difference in the redox distribution between the metal ions and O 2 in iron(III)-superoxo and manganese(IV)-peroxo complexes is rationalized using density functional theory calculations. Metal-dioxygen adducts (M-O 2 ), such as metal-superoxo and metal-peroxo species, are invoked as key intermediates in the transport, storage and activation of dioxygen (O 2 ) by metal-containing proteins and enzymes, as well as in O 2 formation by Photosystem II (refs 1 , 2 , 3 , 4 ). The structures and spectroscopic properties of O 2 -binding metal complexes have been investigated intensively over the past half century and several crystal structures of O 2 -binding iron species have been reported in haem and non-haem iron enzymes and their model compounds [5] , [6] , [7] , [8] , [9] , [10] . One of the first reported crystal structures of an O 2 -bound iron intermediate was obtained using a synthetic haem complex as a model of oxy-haemoglobin and oxy-myoglobin [8] . The structural and spectroscopic characterization of the O 2 -binding iron intermediates in haem-containing proteins and synthetic iron porphyrins revealed that these iron(III)-superoxo species bind the O 2 unit in an end-on manner [7] , [8] , [9] . In contrast, crystal structures of iron-O 2 intermediates in non-haem iron enzymes and models revealed that the O 2 unit in iron(III)-peroxo species binds to the iron centre in a side-on manner [5] , [6] , [10] ; the crystal structure of a mononuclear non-haem iron(III)-peroxo complex, [Fe III (TMC)(O 2 )] + , TMC (1,4,8,11-tetramethyl-1,4,8,11-tetraazacyclotetradecane), shows the binding of O 2 unit in a side-on manner with an O–O bond distance of 1.463(6) Å 10 . Another example is the structure of naphthalene dioxygenase, which shows an O 2 unit bound in a side-on manner [6] . However, to the best of our knowledge, no structural information has been obtained for non-haem iron(III)-superoxo species, although such intermediates have been proposed under catalytic reaction conditions, and trapped and characterized spectroscopically in non-haem iron enzymes and models [11] , [12] , [13] . For example, Nam and colleagues [14] , [15] , [16] proposed the short-lived ‘putative’ Fe(III)-superoxo intermediate during the dioxygen activation by non-haem iron(II) complexes, while Goldberg and colleagues [15] demonstrated that the binding sulfur ligand at the axial position of iron(II) complex facilitated the O 2 binding, therefore generating iron(III)-superoxo species. However, none of these showed direct structural evidence of the iron(III)-superoxo species [14] , [15] , [16] . Further, although non-haem iron(III)-superoxo intermediates have been proposed as reactive species in electrophilic oxidation reactions by non-haem iron complexes, direct evidence for the involvement of such non-haem iron(III)-superoxo species in electrophilic oxidation reactions has not been reported in non-haem iron models [17] , [18] . Furthermore, the involvement of non-haem iron(III)-superoxo species in nucleophilic oxidation reactions has been rarely discussed in either enzymatic or biomimetic reactions. Thus, understanding the structural information and chemical properties, in particular the oxidation reactivity, of iron(III)-superoxo species has become an important objective for bioinorganic chemists. We now report the synthesis, spectroscopic and electronic properties, and crystal structure of a mononuclear side-on ( η 2 ) iron(III)-superoxo complex bearing tetraamido macrocyclic ligand (TAML) [19] , [Fe III (TAML)(O 2 )] 2− ( 1 ). The isolated iron(III)-superoxo complex undergoes both electrophilic and nucleophilic oxidation reactions. In addition, the iron(III)-superoxo complex transfers the bound O 2 unit to a manganese(III) analogue, resulting in the formation of a mononuclear side-on ( η 2 ) manganese(IV)-peroxo complex, [Mn IV (TAML)(O 2 )] 2− ( 2 ). The electronic structures of 1 and 2 are investigated using density functional theory (DFT) calculations to elucidate the difference in the redox distribution between the metal ion and O 2 in these complexes. Synthesis and characterization of 1 The reaction of Na[Fe III (TAML)] with solid potassium superoxide (KO 2 ) in the presence of 6 equiv. of 2.2.2-cryptand in CH 3 CN at 5 °C immediately generated a red intermediate ( 1 ) ( Fig. 1a ; see also Supplementary Fig. 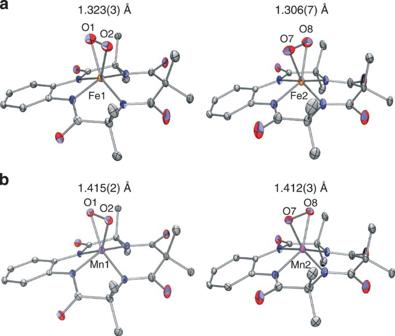Figure 1: X-ray crystal structures of 1 and 2. (a) Displacement ellipsoid plots (30% probability level) of the two crystallographically independent moieties of [FeIII(TAML)(O2)]2−in [K(2.2.2-cryptand)(CH3CN)][K(2.2.2-cryptand)]3-[FeIII(TAML)(O2)]2(see alsoSupplementary Fig. 1andSupplementary Table 1). The O–O bond distances for the two independent moieties are 1.323(3) and 1.306(7) Å, respectively. Disorder of the O7–O8 and the H atoms have been omitted for the sake of clarity. (b) Displacement ellipsoid plots (30% probability level) of the two crystallographically independent moieties of [MnIV(TAML)(O2)]2−in [K(2.2.2-cryptand)(CH3CN)][K(2.2.2-cryptand)]3-[MnIV(TAML)(O2)]2(see alsoSupplementary Fig. 2andSupplementary Table 2). The O–O bond distances for the two independent moieties are 1.415(2) and 1.412(3) Å, respectively. Disorder of the O7–O8 and the H atoms have been omitted for the sake of clarity. 1 and Supplementary Table 1 ), with an electronic absorption band at λ max =490 nm ( ε =2,600 M −1 cm −1 ) ( Fig. 2a and Supplementary Methods ). The intermediate persisted for several days at −20 °C and the greater thermal stability of 1 allowed us to isolate single crystals suitable for structural and spectroscopic analyses, as well as for reactivity studies. The electrospray ionization mass spectrum of 1 exhibits a prominent ion peak at a mass-to-charge ( m/z ) ratio of 873.1, whose mass and isotope distribution pattern correspond to [K(2.2.2-cryptand)Fe(TAML)(O 2 )] − (calculated m/z of 873.3) ( Fig. 2a , inset; also see Supplementary Fig. 3a ). When the reaction was carried out with isotopically labelled K 18 O 2 , a mass peak corresponding to [K(2.2.2-cryptand)Fe(TAML)( 18 O 2 )] − appeared at an m/z of 877.1 (calculated m/z of 877.3). The shift in four mass units on substitution of 16 O with 18 O indicates that 1 contains an O 2 unit ( Fig. 2a , inset). In the electron paramagnetic resonance spectrum of a frozen acetonitrile solution of 1 recorded at 4.3 K, no signal was observed in both perpendicular and parallel modes ( Supplementary Fig. 3b ), which might arise from the electronic configuration of an iron(IV)-peroxo species ( S =1 or 2) or an iron(III) species ( S =1/2, 3/2, or 5/2) coupled with an O 2 − unit of S =1/2. The electronic configuration of 1 was further investigated with 1 H nuclear magnetic resonance Evans method, and the magnetic moment of 3.26 μ B at −20 °C is consistent with an S =1 ground state for 1 . Based on those experimental results, there are three possible structures for 1 : (i) an Fe(IV)-peroxo species with S =1 Fe(IV), (ii) an Fe(III)-superoxo species with S =1/2 Fe(III) ferromagnetically coupled with S =1/2 O 2 − moiety or (iii) an Fe(III)-superoxo species with S =3/2 Fe(III) antiferromagnetically coupled with an S =1/2 O 2 − moiety ( vide infra ). The infrared spectrum of 1 , collected in CH 3 CN at −40 °C, exhibits an isotopically sensitive band at 1,260 cm −1 , which shifts to 1,183 cm −1 on substitution of 16 O with 18 O, consistent with its assignment as an O–O stretching vibration on the basis of the 16–18 Δ value of 77 cm −1 ( 16–18 Δ (calculated)=72 cm −1 ) ( Fig. 2b ). This value is comparable to those recorded for metal-superoxo complexes [9] , [13] , [20] , [21] , suggesting that the O 2 unit in 1 possesses superoxo character. Figure 1: X-ray crystal structures of 1 and 2. ( a ) Displacement ellipsoid plots (30% probability level) of the two crystallographically independent moieties of [Fe III (TAML)(O 2 )] 2− in [K(2.2.2-cryptand)(CH 3 CN)][K(2.2.2-cryptand)] 3 -[Fe III (TAML)(O 2 )] 2 (see also Supplementary Fig. 1 and Supplementary Table 1 ). The O–O bond distances for the two independent moieties are 1.323(3) and 1.306(7) Å, respectively. Disorder of the O7–O8 and the H atoms have been omitted for the sake of clarity. ( b ) Displacement ellipsoid plots (30% probability level) of the two crystallographically independent moieties of [Mn IV (TAML)(O 2 )] 2− in [K(2.2.2-cryptand)(CH 3 CN)][K(2.2.2-cryptand)] 3 -[Mn IV (TAML)(O 2 )] 2 (see also Supplementary Fig. 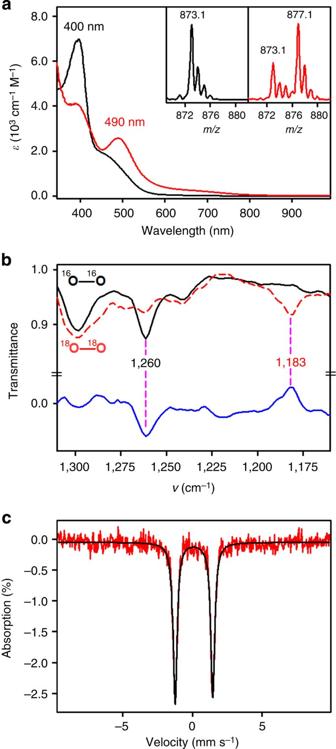Figure 2: Characterization of 1. (a) Ultraviolet–visible spectra of [FeIII(TAML)]−(black line, 0.25 mM) and [FeIII(TAML)(O2)]2−(1, red line, 0.25 mM) in CH3CN at 5 °C. Insets show negative mode electrospray ionization mass spectra of [FeIII(TAML)(16O2)]2−(1-16O2) (black line) and [FeIII(TAML)(18O2)]2−(1-18O2) (red line) obtained in CH3CN at −20°C (see alsoSupplementary Fig. 3bfor a full range of spectrum). (b) Solution infrared spectra of1-16O2(black line, 2.0 mM) and1-18O2(red line, 2.0 mM) in CH3CN at −40 °C. Blue line is a difference spectrum of1-18O2and1-16O2. (c) Mössbauer spectrum of1at 4.2 K in the absence of field.δ=0.096 mm s−1, ΔEq=2.696 mm s−1, consistent with an intermediate-spin Fe(III) centre bound to a TAML ligand. 2 and Supplementary Table 2 ). The O–O bond distances for the two independent moieties are 1.415(2) and 1.412(3) Å, respectively. Disorder of the O7–O8 and the H atoms have been omitted for the sake of clarity. Full size image Figure 2: Characterization of 1. ( a ) Ultraviolet–visible spectra of [Fe III (TAML)] − (black line, 0.25 mM) and [Fe III (TAML)(O 2 )] 2− ( 1 , red line, 0.25 mM) in CH 3 CN at 5 °C. Insets show negative mode electrospray ionization mass spectra of [Fe III (TAML)( 16 O 2 )] 2− ( 1- 16 O 2 ) (black line) and [Fe III (TAML)( 18 O 2 )] 2− ( 1- 18 O 2 ) (red line) obtained in CH 3 CN at −20 ° C (see also Supplementary Fig. 3b for a full range of spectrum). ( b ) Solution infrared spectra of 1- 16 O 2 (black line, 2.0 mM) and 1- 18 O 2 (red line, 2.0 mM) in CH 3 CN at −40 °C. Blue line is a difference spectrum of 1- 18 O 2 and 1- 16 O 2 . ( c ) Mössbauer spectrum of 1 at 4.2 K in the absence of field. δ =0.096 mm s −1 , Δ E q =2.696 mm s −1 , consistent with an intermediate-spin Fe(III) centre bound to a TAML ligand. Full size image Mössbauer spectroscopy was also performed to determine the oxidation state of iron in 1 and define its electronic structure ( Fig. 2c , δ =0.10 mm s −1 and Δ E Q =2.66 mm s −1 ). The isomer shift is in the same range as that for TAML complexes with S =3/2 Fe(III) centres [22] . Following the procedure of Chanda et al . [22] , the density at the nucleus ρ and Δ E Q for this complex were calculated using the 6–311G basis set and B3LYP functional ( Supplementary Methods ); the density at the nucleus was converted into an isomer shift using the calibration of Vrajmasu et al . [23] The computational isomer shift obtained using this method, δ =0.12 mm s −1 , and the calculated Δ E Q , 2.78 mm s −1 , are in excellent agreement with the experimental values. Thus, the spectroscopic data described above suggest that 1 is a mononuclear iron(III) species binding a superoxo ligand, Fe III -O 2 −· . Direct evidence for an Fe–O 2 unit is unambiguously provided from the X-ray crystal structure of 1 , which revealed a mononuclear side-on 1:1 iron complex of O 2 with the triangular Fe–O 2 moiety having a small bite angle (40.37(9)° for O1-Fe1-O2, 39.9(2)° for O7-Fe2-O8 and 39.4(4)° for O7′-Fe2-O8′), which results in a pseudo square pyramidal geometry with side-on biding O 2 moiety ( Fig. 1a , also see Supplementary Fig. 1 and Supplementary Table 1 ). The crystallographically independent O–O bond lengths (O1-O2: 1.323(3) Å, O7-O8/O7′-O8′: 1.306(7)/1.315(12) Å) of 1 are significantly shorter than those of Fe(III)-peroxo species, such as [Fe III (TMC)(O 2 )] + (1.463(6) Å) [10] and naphthalene dioxygenase ( ca . 1.45 Å) [6] , but similar to that of Fe(II)-superoxo species found in homoprotocatechuate 2,3-dioxygenase (1.34 Å) [5] . Further, the observed O–O bond length is close to those of other metal-superoxo complexes that have been characterized structurally ( ca . 1.2–1.3 Å) [9] , [21] . Furthermore, the O 2 ligand within Fe-O 2 unit is almost symmetrically bound to the iron ion with the average Fe–O bond length of 1.927 Å, which is slightly longer than that of [Fe III (TMC)(O 2 )] + (1.910 Å). In accordance with these experimental values, we conclude that 1 is an iron(III)-superoxo complex with the O 2 unit bound in a side-on manner ( η 2 ). To the best of our knowledge, this is the first X-ray crystal structure of a mononuclear non-haem iron(III)-superoxo complex reported in non-haem iron enzyme and model systems. Reactivity studies of 1 As presented in the Introduction section, non-haem iron(III)-superoxo species have attracted much attention recently as active oxidants in a number of enzymatic reactions, especially in electrophilic oxidation reactions by isopenicillin N synthase, myo -inositol oxygenase and cysteine dioxygenase [2] , [24] , [25] . However, nucleophilic reactivity of the non-haem iron(III)-superoxo species has not been previously reported. Moreover, reactivities of synthetic non-haem iron(III)-superoxo complexes in electrophilic and nucleophilic oxidation reactions have been rarely reported in biomimetic studies [20] . We therefore performed these reactions with the isolated, well-characterized non-haem iron(III)-superoxo complex, 1 . First, the reactivity of 1 was examined in the oxidation of C–H and O–H bonds, with precedents that metal-superoxo species are potent oxidants in the C–H and O–H substrate oxygenation reactions [11] , [26] , [27] , [28] . Addition of substrates with weak C–H bonds, such as cyclohexadiene and xanthene, to 1 did not show any spectral changes, indicating that 1 is not capable of activating the C–H bonds of hydrocarbons. In the case of O–H bond activation, addition of 2,4-di- tert -butylphenol to 1 caused the decay of the intermediate with the concurrent formation of [Fe III (TAML)] − ( Supplementary Fig. 4a ). Clear isosbestic points were observed at 333 and 393 nm. The decay rate increased with increase of the substrate concentration, giving a second-order rate constant of 3.0 × 10 −1 M −1 s −1 ( Supplementary Fig. 4b ). Product analysis of the reaction solution revealed the formation of 2,2′-dihydroxy-3,3′,5,5′-tetra- tert -butylbiphenyl as a major product (~75% based on the intermediates used) [29] , [30] . Further, reactions with para -substituted 2,6-di- tert -butylphenols ( p -Y-2,6- t -Bu 2 -C 6 H 2 OH; Y=OMe, Me, H, CN) revealed that the electronegativity of the para -substituents significantly influences the reaction rates ( Supplementary Fig. 5 ); a plot of the relative rates as a function of O–H bond dissociation energies of p -Y-2,6- t -Bu 2 -C 6 H 2 OH shows a good correlation with a slope of –0.65 ( Supplementary Fig. 4c ). In high-valent metal-oxo and metal-superoxo complexes, a linear relationship such as this has been cited in support of an H-atom abstraction mechanism in phenol O–H bond oxidations [29] , [30] , [31] . The nucleophilic reactivity of 1 was investigated in aldehyde deformylation, using 2-phenylpropionaldehyde as a substrate. On addition of 2-phenylpropionaldehyde to 1 in CH 3 CN at 5 °C, 1 was converted to the starting [Fe III (TAML)] − complex with a first-order decay profile ( Supplementary Fig. 6a ) and pseudo-first-order rate constants that increased proportionally with the aldehyde concentration ( k 2 =3.7 M −1 s −1 ) ( Supplementary Fig. 6b ). Product analysis of the resulting solutions revealed the formation of acetophenone (90% based on 1 ), as frequently observed in other nucleophilic oxidation reactions by metal-peroxo complexes [32] , [33] . The reactivity of 1 was further investigated using substituted benzaldehydes with a series of electron-donating and -withdrawing substituents at the para -position of the phenyl group ( para -Y-Ph-CHO; Y=OMe, Me, H, Cl) ( Supplementary Fig. 7 ). A positive ρ + -value of 1.4 in the Hammett plot was obtained ( Supplementary Fig. 6c ), demonstrating that the iron(III)-superoxo complex is an active nucleophilic oxidant; the nucleophilic reactivity of a copper(II)-superoxo complex was reported very recently [34] . To the best of our knowledge, the present results provide the first strong evidence for the involvement of iron(III)-superoxo species in nucleophilic oxidation reactions. The reactivity of 1 was further investigated in an intermolecular O 2 -transfer reaction ( Fig. 3a ), with precedents that metal-peroxo species (for example, [Ni III (12-TMC)(O 2 )] + , [Co III (12-TMC)(O 2 )] + and [Co III (13-TMC)(O 2 )] + ) are capable of transferring their peroxo group to a manganese complex [Mn II (14-TMC)] 2+ to give a manganese-peroxo complex (for example, [Mn III (14-TMC)(O 2 )] + ) [35] , [36] . Interestingly, addition of [Mn III (TAML)] − to a solution containing 1 immediately generated a blue intermediate ( 2 ) ( Fig. 1b ; see also Supplementary Fig. 2 and Supplementary Table 2 ) with an electronic absorption band at 600 nm ( Fig. 3b ); the blue intermediate 2 was characterized as a mononuclear side-on ( η 2 ) manganese(IV)-peroxo complex ( vide infra ). Clear isosbestic points were observed at 462 and 561 nm in the titration reaction ( Fig. 3b and Supplementary Fig. 8 ), in which the O 2 -transfer from 1 to [Mn III (TAML)] − was found to have 1:1 reaction stoichiometry ( Fig. 3b , inset). Kinetic studies of the O 2 -transfer from 1 to [Mn III (TAML)] − were performed in dimethylformamide (DMF) at −20 °C under pseudo-first-order reaction conditions. Addition of 10 equiv. of [Mn III (TAML)] − to the solution of 1 yielded k obs -value of 1.0 × 10 −2 s −1 ( Supplementary Fig. 9a ), with the first-order rate constant increasing proportionally with the concentration of [Mn III (TAML)] − that gives a second-order rate constant ( k 2 ) of 9.0 × 10 −1 M −1 s −1 at –20 °C ( Supplementary Fig. 9b ). The intermolecular O 2 -transfer reaction was dependent on temperature, from which a linear Eyring plot was obtained between −20 °C and 10 °C to give activation parameters of Δ H ‡ =55 kJ mol −1 and Δ S ‡ =−33 J mol −1 K −1 ( Supplementary Fig. 10 ). The temperature dependence of the rate constants and the significant negative entropy value suggest that a bimolecular mechanism is operating in the O 2 -transfer reaction, where the formation of a presumed [(TAML)Fe-O 2 -Mn(TAML)] 3− intermediate is the rate-determining step [35] , [36] . Finally, the reverse reaction, which is the O 2 -transfer from 2 to [Fe III (TAML)] − to form [Mn III (TAML)] − and 1 , does not occur. 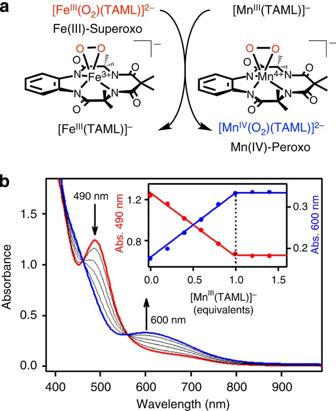Figure 3: O2-transfer reaction of 1. (a) A reaction scheme showing O2-transfer from [FeIII(TAML)(O2)]2−(1) to [MnIII(TAML)]−that results in the formation of [FeIII(TAML)]−and [MnIV(TAML)(O2)]2−(2). (b) Ultraviolet–visible spectral changes showing the formation of2(blue line) and the disappearance of1(red line) on addition of [MnIII(TAML)]−to1in increments of 0.2 equiv. in dimethylformamide at −20 °C. Inset shows the spectroscopic titration at 490 nm (red circle) for the decay of1and 600 nm (blue circle) for the formation of2as a function of the equivalents of [MnIII(TAML)]–added to1. Figure 3: O 2 -transfer reaction of 1. ( a ) A reaction scheme showing O 2 -transfer from [Fe III (TAML)(O 2 )] 2− ( 1 ) to [Mn III (TAML)] − that results in the formation of [Fe III (TAML)] − and [Mn IV (TAML)(O 2 )] 2− ( 2 ). ( b ) Ultraviolet–visible spectral changes showing the formation of 2 (blue line) and the disappearance of 1 (red line) on addition of [Mn III (TAML)] − to 1 in increments of 0.2 equiv. in dimethylformamide at −20 °C. Inset shows the spectroscopic titration at 490 nm (red circle) for the decay of 1 and 600 nm (blue circle) for the formation of 2 as a function of the equivalents of [Mn III (TAML)] – added to 1 . Full size image In this section, we have shown that the non-haem iron(III)-superoxo complex, 1 , is an active oxidant in both electrophilic and nucleophilic reactions. We have also shown that the O 2 unit in the iron(III)-superoxo complex is transferred to a Mn(III) complex. Detailed mechanistic studies are underway to understand the chemical properties and mechanisms of non-haem iron(III)-superoxo species in oxidation reactions. Synthesis and characterization of 2 The manganese(IV)-peroxo complex, [Mn IV (TAML)(O 2 )] 2− ( 2 ), was synthesized independently by reacting Li[Mn III (TAML)] with solid KO 2 in the presence of 6 equiv. of 2.2.2-cryptand in CH 3 CN at 25 °C (see Supplementary Figs 11 and 12 , and Supplementary Table 3 for the spectroscopic and structural characterization of [Mn III (TAML)] − ). The high stability of 2 at room temperature allowed us to isolate single crystals suitable for structural and spectroscopic characterization. The ultraviolet–visible spectrum of 2 exhibits an absorption band at 600 nm ( ε =720 M −1 cm −1 ) ( Supplementary Fig. 13a ). The electrospray ionization mass spectrum of 2 exhibits a prominent ion peak at a mass-to-charge ( m/z ) ratio of 872.1 and its isotopic distribution pattern was in good agreement with [K(2.2.2-cryptand)Mn(TAML)( 16 O 2 )] − (calculated m/z of 872.3) ( Supplementary Fig. 13b ). When 2 was prepared with isotopically labelled K 18 O 2 , a mass peak corresponding to [K(2.2.2-cryptand)Mn(TAML)( 18 O 2 )] − appeared at a m/z of 876.1 (calculated m/z of 876.3). The shift in four mass units on substitution of 16 O with 18 O indicates that 2 contains an O 2 unit ( Supplementary Fig. 13b , inset). The electron paramagnetic resonance spectrum of 2 exhibits one six-line hyperfine pattern centred at g =5.6 with splitting of a =55 G and two broad signals at g =2.3 and 1.7, indicating an S =3/2 Mn(IV) ground state ( Supplementary Fig. 13c ) [37] , [38] . The solid infrared spectrum (KBr) of 2 exhibits an isotopically sensitive band at 905 cm –1 , which shifts to 860 cm −1 on substitution of 16 O with 18 O 2 , consistent with its assignment as an O–O stretching vibration on the basis of the 16–18 Δ value of 45 cm −1 ( 16–18 Δ (calculated)=52 cm −1 ) ( Supplementary Fig. 14 ). This value is comparable to those recorded for metal-peroxo complexes [38] , [39] , thus leading us to conclude that the O 2 unit in 2 possesses peroxo character. The X-ray crystal structure of 2 is given in Fig. 1b (also see Supplementary Fig. 2 and Supplementary Table 3 ). Although complex 2 also contains a mononuclear side-on, 1:1 Mn–O 2 moiety best described as a pseudo square pyramidal geometry with small acute angles of 44.30(7)° for O1-Mn1-O2, 44.17(11)° for O7-Mn2-O8 and 43.9(4)° for O7′-Mn2-O8′ ( Supplementary Fig. 2 ). By comparison with the structure of 1 , the O–O bond distances in 2 are significantly different. Contrary to the shorter O–O bond length of 1 determined by the X-ray crystal structure, the crystallographically independent O–O bond distances for 2 are 1.415(2) (O1-O2), 1.412(3) (O7-O8) and 1.403(13) (O7′-O8′) Å, which are significantly longer than 1 and even longer than recently reported O–O bond distance of a mononuclear non-haem Mn(IV)-peroxo (1.379(3) Å) complex [38] . The average Mn–O distance of 1.876 Å is within the range of 1.841–1.901 Å for the monomeric side-on Mn(III)-peroxo complexes [33] . Moreover, this mean value is close to that of Mn(IV)-peroxo (1.878(2) Å) supported by tetradentate trianionic ligand [38] . Taken together, the spectroscopic and structural data unambiguously demonstrate that 2 is a high-spin ( S =3/2) Mn(IV)-peroxo complex binding the O 2 2− unit in a side-on manner ( η 2 ). Computational studies of 1 and 2 To elucidate the electronic structures of 1 and 2 , DFT geometry optimizations were carried out on each complex starting from the atomic coordinates refined in both crystal structures and using its experimental spin state. For 1 , a series of functionals employing varying amounts of Hartree–Fock exchange were used (BP86 (0%), TPSSh (10%), B3LYP (20%), BP86+25% Hartree-Fock exchange and M06 (27%)), all with the TZVP basis set. 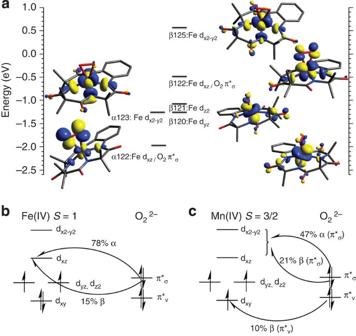Figure 4: DFT calculations on 1 and electronic structures for 1 and 2. (a) Unoccupied MOs for1with significant Fe or O2π* character. (b) Derived from the MOs presented ina, which show 78% delocalization of theα π*σelectron and 15% delocalization of theβ π*σelectron from O2into the unoccupied Fedxzorbital, leading to significantS=3/2 Fe(III) antiferromagnetically coupled toS=1/2 O2character. (c) Derived from the MOs presented inSupplementary Fig. 16. The BP86 functional with 25% Hartree–Fock exchange gives an optimized structure most consistent with the crystallographic data ( Supplementary Table 4 for geometric parameters). Note from Supplementary Table 4 that the O–O distance is most sensitive to functional and the experimental 1.32 Å distance, which reflects the amount of charge transfer from the metal to O 2 , and is best reproduced by this hybrid functional (although M06 also gives a good O–O distance, its average Fe–O bond length is too long). For 2 , the geometry optimization results using the BP86, TPSSh, B3LYP and M06 functionals were compared, and the closest agreement with the experimental O–O bond length was obtained using B3LYP ( Supplementary Table 5 ). As it was necessary to use BP86+25% Hartree-Fock exchange to reproduce the structure of 1 , the Mössbauer parameters were recalculated using this functional (see Supplementary Fig. 15 for the calibration of experimental isomer shifts with calculated ρ at the Fe). The isomer shift obtained of δ =0.11 mm s −1 is again consistent with the experimental value of 0.10 mm s −1 . As the DFT-derived geometry-optimized structures for 1 and 2 give reasonable agreement with the experimental data, their associated electronic structures were evaluated. The unoccupied orbitals calculated for 1 with significant Fe d or O 2 π * character are displayed in Fig. 4a (the unoccupied orbitals reflect the uncompensated electron density in the occupied orbitals). From Fig. 4a , the electronic structure of 1 lies between the limits of an S =1 Fe(IV)-peroxo and an S =3/2 Fe(III) antiferomagnetically coupled to an S =1/2 superoxo species. The Mülliken population analysis of the unoccupied orbitals shows 78% O 2 π * σ character (where π * σ is the in-[Fe-O 2 ]-plane π * orbital on O 2 ; π * v is out-of-plane) in the α -unoccupied d xz orbital and 15% O 2 π * σ character in the β -unoccupied d xz orbital. From the Fe(IV)-peroxo limit, this is consistent with significant delocalization of an O 2 2− electron onto the Fe and is thus closer to the Fe(III)-superoxo limit ( Fig. 4b ). The low-energy unoccupied π * σ character on the superoxo is consistent with its H-atom abstraction reactivity. Similarly, for the calculated electronic structure of 2 , starting from the Mn(IV)-peroxo limit, the unoccupied orbitals ( Supplementary Fig. 16 ) show delocalization of α and β O 2 2− π * σ electrons (47% and 21%, respectively) into the unoccupied Mn d xz orbital, in addition to 10% delocalization of the β O 2 2− π * v electron into the β-unoccupied d xy orbital (which is occupied in 1 ) ( Fig. 4c ). This gives a total delocalization of 78% of a O 2 2− π * electron onto the Mn, less than the delocalization onto Fe in 1 (93%), which places 2 closer to the Mn(IV)-peroxo limit, consistent with the longer O–O bond length in 2 . Figure 4: DFT calculations on 1 and electronic structures for 1 and 2. ( a ) Unoccupied MOs for 1 with significant Fe or O 2 π * character. ( b ) Derived from the MOs presented in a , which show 78% delocalization of the α π * σ electron and 15% delocalization of the β π * σ electron from O 2 into the unoccupied Fe d xz orbital, leading to significant S =3/2 Fe(III) antiferromagnetically coupled to S =1/2 O 2 character. ( c ) Derived from the MOs presented in Supplementary Fig. 16 . Full size image To understand the differences between the geometric and electronic structures of 1 and 2 , an extra electron was added to each complex and the ionization energy of these hypothetical M(III)(TAML)-peroxo complexes was calculated, using the possible initial spin states ( S =3/2 for Fe III , S =1 and 2 for Mn III ) and the final spin states observed experimentally for 1 ( S =1) and 2 ( S =3/2). This evaluates whether there is a difference in the reduction potential between these metal ions in this ligand set. The results of these calculations are summarized in Supplementary Table 6 , along with those of parallel calculations with a redox-innocent Cl − ligand in place of the peroxide. Relative to the iron complex, ionization of an electron from a hypothetical S =1 Mn(III)-O 2 2− is easier by 0.42 eV (1.23 eV with the Cl − ligand), while ionization of an electron from an S =2 Mn(III)-O 2 2− is approximately isoenergetic. From Fig. 4c and Supplementary Fig. 16 , the electronic structure of 2 has significant S =1 Mn(III) character. These calculations indicate that the reduction potential of the metal centre in the MnO 2 complex is lower than that of the metal centre in the FeO 2 complex, consistent with increased electron density donation from the peroxide in 1 that results in significant Fe(III)-superoxo character relative to 2 . In summary, we have reported the first synthetic mononuclear non-haem iron(III)-superoxo complex and a manganese(IV)-peroxo complex bearing a common supporting ligand. The crystal structures of those intermediates determined via single crystal X-ray crystallography demonstrate unambiguously that the O 2 units in the iron(III)-superoxo and manganese(IV)-peroxo complexes are bound to the iron and manganese ions in a side-on manner. The difference in electron distribution between the metal and the O 2 reflects the higher reduction potential of the Fe(III). The non-haem iron(III)-superoxo complex undergoes both electrophilic and nucleophilic oxidation reactions. This model study suggests that both reactivities might be important in non-haem iron enzyme catalysis, which remains to be evaluated. How to cite this article: Hong, S. et al . Crystallographic and spectroscopic characterization and reactivities of a mononuclear non-haem iron(III)-superoxo complex. Nat. Commun. 5:5440 doi: 10.1038/ncomms6440 (2014). Accession codes: The X-ray crystallographic coordinates for structures reported in this Article have been deposited at the Cambridge Crystallographic Data Centre (CCDC), under deposition number CCDC 1001933–1001935. These data can be obtained free of charge from The Cambridge Crystallographic Data Centre via www.ccdc.cam.ac.uk/data_request/cif .